Electronic origin of high-temperature superconductivity in single-layer FeSe superconductor The recent discovery of high-temperature superconductivity in iron-based compounds has attracted much attention. How to further increase the superconducting transition temperature ( T c ) and how to understand the superconductivity mechanism are two prominent issues facing the current study of iron-based superconductors. The latest report of high- T c superconductivity in a single-layer FeSe is therefore both surprising and significant. Here we present investigations of the electronic structure and superconducting gap of the single-layer FeSe superconductor. Its Fermi surface is distinct from other iron-based superconductors, consisting only of electron-like pockets near the zone corner without indication of any Fermi surface around the zone centre. Nearly isotropic superconducting gap is observed in this strictly two-dimensional system. The temperature dependence of the superconducting gap gives a transition temperature T c ~ 55 K. These results have established a clear case that such a simple electronic structure is compatible with high- T c superconductivity in iron-based superconductors. The latest report of high-temperature superconductivity signature in single-layer FeSe [1] is significant because it is possible to break the superconducting transition temperature record (maximum T c ~55 K) that has been stagnant since the discovery of the iron-based superconductors in 2008 [2] , [3] , [4] , [5] , [6] . Such a high T c is unexpected in the FeSe system, because the bulk FeSe exhibits a T c of only 8 K at ambient pressure [5] , although it can be enhanced to 36.7 K under high pressure [7] . The T c is still unusually high, even considering the newly discovered intercalated FeSe system A x Fe 2 −y Se 2 (A=K, Cs, Rb and Tl) with a T c of 32 K at ambient pressure [8] , [9] and possible T c near 48 K under high pressure [10] . Understanding the origin of high-temperature superconductivity in such a two-dimensional (2D) FeSe system is crucial to understanding the superconductivity mechanism in the Fe-based superconductors in particular, and providing key insights on how to achieve high-temperature superconductivity in general. As the physical properties and superconductivity of a material are dictated by its underlying electronic structure, it is essential to carry out such investigations on the high T c single-layer FeSe superconductor that shows advantages in a number of aspects. First, among the Fe-based superconductors discovered so far [2] , [3] , [4] , [5] , [6] , FeSe superconductor has the simplest crystal structure consisting only of FeSe layer that is considered to be the essential building block for superconductivity in the Fe-based compounds [5] . Second, single-layer FeSe, composed of a Se–Fe–Se stack along the c axis with a thickness of 5.5 Å, is a strictly 2D system. This gives rise to a 2D electronic structure without complications of k z momentum along the c direction. To obtain a complete electronic structure and to pin down a gap node in the superconducting state, one has to exhaust all the three-dimensional (3D) momentum space that is usually difficult in typical 3D bulk superconductors [11] . Third, the FeSe superconductor is an ideal system where the superconducting phase is pure and well characterized. This is in contrast to the A x Fe 2− y Se 2 (A=K, Cs, Rb, Tl and etc.) superconducting system [8] , [9] , [12] where there exists phase inhomogeneity and the real superconducting phase remains not clearly identified. Most importantly, the discovery of high- T c superconductivity in the single-layer FeSe [1] provides a venue to sort out the key components in achieving high-temperature superconductivity in the Fe-based compounds. Here we report detailed investigation of electronic structure and superconducting gap in the single-layer FeSe superconductor by high-resolution angle-resolved photoemission spectroscopy (ARPES) measurements. Its Fermi-surface topology is distinct from other Fe-based superconductors. It consists only of electron-like pockets near the zone corner without indication of any Fermi surface around the zone centre. We observed nearly isotropic superconducting gap around the Fermi surface; it rules out the existence of gap node in this 2D system. Detailed temperature dependence of the superconducting gap gives a superconducting transition temperature of T c ~55 K. These results indicate that such a simple distinct Fermi-surface topology is compatible with the occurrence of high-temperature superconductivity in the Fe-based superconductors. They will shed lights on understanding the superconductivity mechanism and exploring new superconductors with higher T c in the Fe-based superconductors. 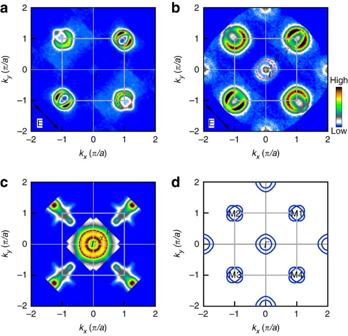Figure 1: Fermi surface of the single-layer FeSe superconductor. (a) Fermi-surface mapping of single-layer FeSe measured at 20 K that consists only of the electron-like Fermi-surface sheet (γ) aroundM(π,π). (b) Fermi-surface mapping of (Tl,Rb)xFe2−ySe2superconductor (Tc=32 K) that consists of electron-like Fermi-surface sheet (γ) aroundMand also electron-like Fermi-surface sheets (αandβ) aroundΓ(0,0)14. (c) Fermi-surface mapping of (Ba1.6K0.4)Fe2As2superconductor (Tc=35 K) that consists of hole-like Fermi-surface sheets (αandβ) aroundΓand complex Fermi surface nearMregion17. The spectral weight near the second zone centres is absent because the measured region did not cover this area. (d) Fermi surface ofβ-FeSe by band-structure calculations forkz=0 (blue thick lines) that consists of hole-like Fermi-surface sheets aroundΓand two electron-like Fermi-surface sheets aroundM(ref.21). For convenience, the four equivalentMpoints are labelled asM1(π,π),M2(−π,π),M3(−π,−π) andM4(π,−π). Fermi surface and band structure Figure 1a shows Fermi-surface mapping of the single-layer FeSe thin film covering multiple Brillouin zones. In comparison, we also present Fermi surface of (Tl,Rb) x Fe 2 −y Se 2 superconductor ( T c =32 K) ( Fig. 1b ) [13] , [14] , [15] , [16] and (Ba 1.6 K 0.4 )Fe 2 As 2 ( T c =35 K)( Fig. 1c ) [17] , [18] , [19] , [20] , as well as the Fermi surface of FeSe by band-structure calculations ( Fig. 1d ) [21] . The band structure along some typical cuts ( Fig. 2d ) are shown in Fig. 2a,c . The photoemission spectra (energy distribution curves, EDCs) corresponding to Fig. 2a are shown in Fig. 2b . For the single-layer FeSe superconductor, we only observe a clear electron-like Fermi surface around M ( π , π )(denoted as γ hereafter) ( Fig. 1a ) but do not observe any indication of Fermi surface around the Γ (0,0) point. The γ Fermi surface is nearly circular; the corresponding Fermi momentum ( k F ) for the cut crossing the M point ( Fig. 2a ) is approximately 0.25 in a unit of π / a (lattice constant a =3.90 Å) that is significantly smaller than 0.35 π / a found in (Tl,Rb) x Fe 2− y Se 2 superconductor [14] . Considering that the Fermi surface around M consists of two degenerate Fermi-surface sheets ( Fig. 1d ), this yields an electron counting of about 0.10 electrons/Fe. This is considerably smaller than that in (Tl,Rb) x Fe 2− y Se 2 superconductor (0.18 electrons per Fe when only considering the M point electron Fermi-surface sheets). This value in the single-layer FeSe superconductor is closer to the optimal doping level in electron-doped Ba(Fe 1− x Co x )As 2 ( x ~0.07) system [22] . On the other hand, the γ band bottom in single-layer FeSe lies at 60 meV below the Fermi level, slightly deeper than the 50 meV in (Tl,Rb) x Fe 2− y Se 2 superconductor [14] . The Fermi-surface size and the bandwidth together give an effective electron mass of 2.7 m e (m e is free electron mass) in the single-layer FeSe and 6.1 m e in (Tl,Rb) x Fe 2− y Se 2 superconductor. This indicates that in single-layer FeSe, the electrons are lighter than those in (Tl,Rb) x Fe 2− y Se 2 superconductor, possibly related to a weaker electron correlation. Figure 1: Fermi surface of the single-layer FeSe superconductor. ( a ) Fermi-surface mapping of single-layer FeSe measured at 20 K that consists only of the electron-like Fermi-surface sheet ( γ ) around M ( π , π ). ( b ) Fermi-surface mapping of (Tl,Rb) x Fe 2−y Se 2 superconductor ( T c =32 K) that consists of electron-like Fermi-surface sheet ( γ ) around M and also electron-like Fermi-surface sheets ( α and β ) around Γ (0,0) [14] . ( c ) Fermi-surface mapping of (Ba 1.6 K 0.4 )Fe 2 As 2 superconductor ( T c =35 K) that consists of hole-like Fermi-surface sheets ( α and β ) around Γ and complex Fermi surface near M region [17] . The spectral weight near the second zone centres is absent because the measured region did not cover this area. ( d ) Fermi surface of β -FeSe by band-structure calculations for k z =0 (blue thick lines) that consists of hole-like Fermi-surface sheets around Γ and two electron-like Fermi-surface sheets around M (ref. 21 ). For convenience, the four equivalent M points are labelled as M 1( π , π ), M 2(− π , π ), M 3(− π ,− π ) and M 4( π ,− π ). 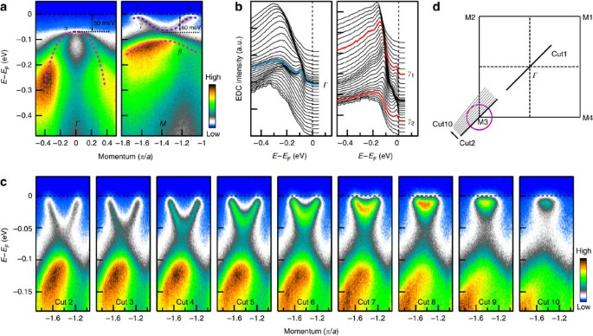Figure 2: Band structure and photoemission spectra of the single-layer FeSe superconductor. (a) Band structure along the cut 1 crossing theΓpoint (left panel) and along the cut 2 crossing theM3 point (right panel). The pink dashed line in the left panel shows schematically a hole-like band near theΓpoint with its top at 80 meV below the Fermi level. The purple dashed line in the right panel shows schematically an electron-like band with its bottom at 60 meV below the Fermi level. (b) Photoemission spectra (EDCs) corresponding to image (a) for the cut 1 (left panel) and the cut 2 (right panel). The blue line in left panel corresponds to EDC atΓpoint whereas the two red curves in right panel correspond to EDCs at two Fermi momenta (γ1andγ2of the electron-like band nearM. (c) Detailed band-structure evolution near theM3 region from the cut 2 (left-most panel) to the cut 10 (right-most panel). (d) The location of the momentum cuts along some high-symmetry lines and near theM3 region. Full size image Figure 2: Band structure and photoemission spectra of the single-layer FeSe superconductor. ( a ) Band structure along the cut 1 crossing the Γ point (left panel) and along the cut 2 crossing the M 3 point (right panel). The pink dashed line in the left panel shows schematically a hole-like band near the Γ point with its top at 80 meV below the Fermi level. The purple dashed line in the right panel shows schematically an electron-like band with its bottom at 60 meV below the Fermi level. ( b ) Photoemission spectra (EDCs) corresponding to image ( a ) for the cut 1 (left panel) and the cut 2 (right panel). The blue line in left panel corresponds to EDC at Γ point whereas the two red curves in right panel correspond to EDCs at two Fermi momenta ( γ 1 and γ 2 of the electron-like band near M . ( c ) Detailed band-structure evolution near the M 3 region from the cut 2 (left-most panel) to the cut 10 (right-most panel). ( d ) The location of the momentum cuts along some high-symmetry lines and near the M 3 region. Full size image The observation of only electron-like Fermi-surface sheets around M makes the single-layer FeSe superconductor distinct from all the other Fe-based superconductors. Most of the Fe-based superconductors, such as (Ba,K)Fe 2 As 2 , are characterized by hole-like Fermi-surface sheets around the Γ point according to band-structure calculations [23] , [24] and ARPES measurements( Fig. 1c ) [17] , [18] , [19] , [20] . It is also different from the Fermi-surface topology of the recently discovered A x Fe 1− y Se 2 superconductors, where the Fermi-surface sheets remain present around the Γ point ( Fig. 1b ), although all observed Fermi-surface sheets are exclusively electron-like [13] , [14] , [15] , [16] . The 2D nature of the single-layer FeSe also removes any ambiguity of the possible k z complications that are common in other Fe-based systems. We note that, compared with the band structure of (Tl,Rb) x Fe 2− y Se 2 superconductor, the band structure of single-layer FeSe is not a simple rigid band shift. First, as mentioned above, the γ band shape near M is significantly different leading to a lighter effective mass. Second, the much lower electron doping in FeSe superconductor is expected to shift the bands towards the Fermi level when comparing with the bands in (Tl,Rb) x Fe 2− y Se 2 superconductor. However, the top of the hole-like α band near Γ point in FeSe superconductor ( Fig. 2a , left panel, 80 meV below the Fermi level) is similar to that in (Tl,Rb) x Fe 2− y Se 2 superconductor [14] . The bottom of the electron-like γ band near M in FeSe ( Fig. 2a , right panel, 60 meV below the Fermi level) is even deeper than that in (Tl,Rb) x Fe 2−y Se 2 superconductor (~50 meV below the Fermi level) [14] , which is in opposite direction from expectation. Superconducting gap The identification of clear γ Fermi-surface sheet near M point makes it possible to investigate the superconducting gap in this new superconductor. We start first by examining the temperature dependence of the superconducting gap. 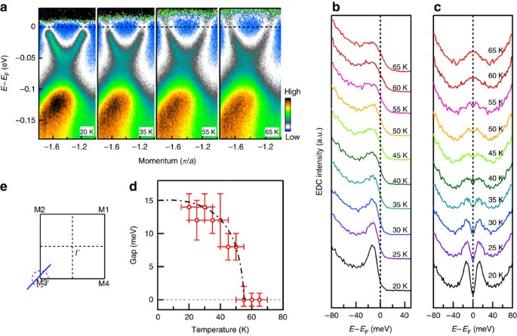Figure 3: Temperature dependence of superconducting gap of the single-layer FeSe superconductor. (a) Typical photoemission images along the momentum cut near theM3 point (blue line in (e)) measured at different temperatures. The temperature labelled here is a usual nominal sample temperature (see 'sample temperature calibration' in Methods). Each image is divided by the corresponding Fermi distribution function to highlight opening or closing of an energy gap. (b) Photoemission spectra at the Fermi crossings ofγFermi surface and their corresponding symmetrized spectra (c) measured at different temperatures. (d) Temperature dependence of the superconducting gap. The error bars are defined as s.d. The dashed line is a BCS gap form that gives a gap size of 15 meV at zero temperature. (e) Location of the momentum cut nearM3 point (blue line). The dashed shows schematically the electron-like Fermi-surface nearMpoint. Figure 3a shows the photoemission images along the cut near M 3 (its location shown in Fig. 3e ) at different temperatures. The corresponding photoemission spectra (EDCs) on the Fermi momentum are shown in Fig. 3b, where sharp peaks develop at low temperatures. To visually inspect possible gap opening and remove the effect of Fermi distribution function near the Fermi level, these original EDCs are symmetrized ( Fig. 3c ), following the procedure commonly used in the study of high-temperature cuprate superconductors [25] . For the γ pocket near M , there is a clear gap opening at low temperature (20 K), as indicated by a dip at the Fermi energy in the symmetrized EDCs ( Fig. 3c ). With increasing temperature, the dip at E F is gradually filled up and is almost invisible near 50–55 K. As it is commonly observed from ARPES on the Fe-based superconductors that the gap closes at the superconducting temperature [17] , [14] , Fig. 3c suggests that the single-layer FeSe sample, we measured, has a T c around (55±5 K) (see 'sample temperature calibration' in Methods). This value is reproducible with an independent measurement on another sample. The temperature dependence of the superconducting gap size ( Fig. 3d ) follows the form of the BCS theory of superconductivity. Due to technical difficulties, it is not yet possible to directly measure superconducting transition temperature on the single-layer FeSe thin film by transport or magnetic measurements [1] . The gap size measured at 20 K is ~15 meV. As a high-resolution ARPES measurement on (Tl,Rb) x Fe 2− y Se 2 superconductor ( T c =32 K) gives a superconducting gap of ~9.7 meV [12] , if we assume the same ratio between the superconducting gap size and T c , 15 meV gap in the single-layer FeSe would correspond to ~50 K that is consistent with the value from the temperature-dependent gap measurement. Figure 3: Temperature dependence of superconducting gap of the single-layer FeSe superconductor. ( a ) Typical photoemission images along the momentum cut near the M 3 point (blue line in ( e )) measured at different temperatures. The temperature labelled here is a usual nominal sample temperature (see 'sample temperature calibration' in Methods). Each image is divided by the corresponding Fermi distribution function to highlight opening or closing of an energy gap. ( b ) Photoemission spectra at the Fermi crossings of γ Fermi surface and their corresponding symmetrized spectra ( c ) measured at different temperatures. ( d ) Temperature dependence of the superconducting gap. The error bars are defined as s.d. The dashed line is a BCS gap form that gives a gap size of 15 meV at zero temperature. ( e ) Location of the momentum cut near M 3 point (blue line). The dashed shows schematically the electron-like Fermi-surface near M point. Full size image Now, we come to the momentum-dependent measurements of the superconducting gap. For this purpose, we took high-resolution Fermi-surface mapping (energy resolution of 4 meV) of the γ pocket at M ( Fig. 4d ). 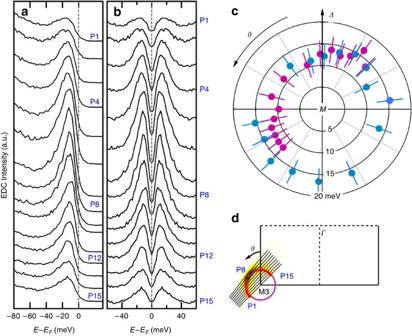Figure 4: Momentum dependence of superconducting gap of the single-layer FeSe superconductor. (a) EDCs along theγFermi surface and (b) their corresponding symmetrized EDCs measured at 20 K. (c) Momentum dependence of the superconducting gap, obtained by picking the peak position in the symmetrized EDCs, along theγFermi surface. Two superconducting samples are independently measured and their superconducting gaps are both shown with the pink solid circles representing the gap of sample #1 and the blue solid circles representing the gap of sample #2. The error bars are defined as s.d. (d) The Fermi-surface mapping nearM3 and the corresponding Fermi crossings for sample #1. The violet circle represents the Fermi surface. The red solid circles represent measured Fermi momenta that are labelled as P1 to P15 (for clarity, the intermittent points are not labelled). The labels in (a) and (b) correspond to the Fermi momentum labels in (d). Figure 4a shows photoemission spectra (EDCs) around the γ Fermi surface measured in the superconducting state ( T = 20 K); the corresponding symmetrized photoemission spectra are shown in Fig. 4b . We have carried out two independent measurements on two samples; the extracted superconducting gap for both samples is nearly isotropic. The sample #1 shows a superconducting gap with a size of (13±2) meV whereas the other sample #2 has a gap of (15±2) meV. We note that superconductivity in single-layer FeSe is sensitive to the preparation and post-annealing conditions. The slight difference in the gap size is possibly due to slightly different post-annealing conditions that caused a subtle variation of the superconducting phase. In both samples, no indication of zero gap is observed around the γ Fermi surface. Since the measured single-layer FeSe is strictly 2D in nature, it avoids complications from 3D Fermi surface associated with bulk materials. This establishes unambiguously that there is no node in the superconducting gap ( Fig. 4c ). Figure 4: Momentum dependence of superconducting gap of the single-layer FeSe superconductor. ( a ) EDCs along the γ Fermi surface and ( b ) their corresponding symmetrized EDCs measured at 20 K. ( c ) Momentum dependence of the superconducting gap, obtained by picking the peak position in the symmetrized EDCs, along the γ Fermi surface. Two superconducting samples are independently measured and their superconducting gaps are both shown with the pink solid circles representing the gap of sample #1 and the blue solid circles representing the gap of sample #2. The error bars are defined as s.d. ( d ) The Fermi-surface mapping near M 3 and the corresponding Fermi crossings for sample #1. The violet circle represents the Fermi surface. The red solid circles represent measured Fermi momenta that are labelled as P1 to P15 (for clarity, the intermittent points are not labelled). The labels in ( a ) and ( b ) correspond to the Fermi momentum labels in ( d ). Full size image Although the observed Fermi-surface topology and nearly isotropic nodeless superconducting gap seem to be reminiscent to that of A x Fe 2− y Se 2 superconductors [13] , [14] , [15] , [16] , their revelation in the single-layer FeSe system with high T c provides much profound and decisive information on understanding the physics and superconductivity mechanism of Fe-based superconductors. First, in the newly discovered A x Fe 2− y Se 2 superconductors, because of the coexistence of many different phases, it remains controversial on which phase is truely superconducting [12] . The single-layer FeSe system provides a clear-cut case that the Fe-vacancy-free FeSe phase can support high-temperature superconductivity. Second, the complete absence of Fermi surface around the Γ point removes any scattering channel between the Γ Fermi surface sheet and M -point Fermi surface sheet. This makes it more straightforward than that in A x Fe 2− y Se 2 superconductors where Fermi surface sheets are still present around Γ point albeit being electron-like. Third, because of the 2D nature of the single-layer FeSe, the present observation can make a straightforward conclusion that the superconducting gap is nearly isotropic and nodeless. In 3D A x Fe 2− y Se 2 superconductors, such a conclusion cannot be made unambiguously before one carries out measurements for the entire momentum space along all k z (ref. 11 ). The present work has important implications on the pairing mechanism in Fe-based superconductors. The electronic structure of the Fe-based compounds involves all five Fe 3d -orbitals forming multiple Fermi-surface sheets: hole-like Fermi-surface sheets around Γ and electron-like ones around M (refs 23 , 24 ). It has been proposed that the interband scattering between the hole-like bands near Γ and the electron-like bands near M is responsible for electron pairing and superconductivity [24] , [26] , [27] , [28] , [29] , [30] , [31] . The absence of Fermi surface around Γ point in the single-layer FeSe superconductor, with the top of the hole-like band lying well below the Fermi level (80 meV below E F , Fig. 2a , left panel), completely rules out the electron scattering possibility across the Fermi-surface sheets between the Γ and M points. Furthermore, with the absence of Fermi surface around Γ , electrons can only scatter across the Fermi-surface sheets between M points that is predicted to result in d -wave superconducting gap [24] , [32] , [33] , [34] . It is argued that two Fermi-surface sheets around a given M point with opposite phases can give rise to gap nodes around the Fermi surface [35] . In this case, our identification of nodeless superconducting gap does not favour such a scheme of electron scattering across M -point Fermi-surface sheets as the pairing mechanism in the Fe-based superconductors. This is in contrast to the low- T c FeSe case ( T c =8 K) where there is a clear indication of nodes in the superconducting gap [36] . Other alternative pictures, such as the interaction of local Fe-magnetic moment [37] , [38] , [39] , [40] , [41] ,or orbital fluctuations [42] , [43] , need to be invoked to understand high-temperature superconductivity in the single-layer FeSe superconductor. There are a couple of intriguing issues that merit further investigations. First, there is a disagreement between the previous tunnelling measurements [1] and our present ARPES measurements. Although two peaks at 20.1 meV and 9.0 meV are developed in the tunnelling spectrum in the superconducting state of a single-layer FeSe superconductor [1] , the present ARPES measurements do not reveal the two-gap structure in the momentum-resolved spectra. The maximum superconducting gap (~15 meV) in our measurement is smaller than 20.1 meV but larger than 9.0 meV. Moreover, with the identification of only one Fermi surface near M , and a nearly isotropic superconducting gap, the observation of two gaps can not be explained by multiple gaps on different Fermi-surface sheets, as found in other Fe-based supercouductors like (Ba,K)Fe 2 Se 2 (refs 17 , 18 ). As tunnelling is a local probe, it is highly unlikely to attribute these two peaks as due to phase separation on such a small scale. Although we are carrying out experiment to ensure that there is no change in the sample during the de-capping process of the amorphous Se protection-layer in ARPES experiment, one conjecture is whether both the FeSe thin film and the interface between FeSe and SrTiO 3 may become superconducting with different gap sizes. This comes to another prominent issue whether the observed superconductivity is due to FeSe itself or the interface between the FeSe and the SrTiO 3 substrate. The main electronic feature of electron-like γ Fermi surface is consistent with the band-structure calculations of FeSe, and the energy gap on this particular Fermi surface closes at high temperature. Also, we do not see signature of possible 2D electron gas in the interface as no electron-like Fermi surface around the Γ point is observed. These observations seem to favour the attribution of superconductivity to the FeSe layer. Because the lattice constant for bulk FeSe is a =3.76 Å (ref. 5 ) and for SrTiO 3 is a =3.905 Å, an apparent lattice mismatch between FeSe and SrTiO 3 is expected to exert a strong tensile strain on the FeSe layer when FeSe is epitaxially grown on SrTiO 3 (001) substrate. Such a tensile pressure on FeSe layer may have an important role, as it has been shown that superconductivity in FeSe is rather sensitive to high pressure [7] , [10] . However, we cannot fully rule out interface superconductivity, when considering FeSe, may become superconducting owing to the proximity effect and weak signal from the buried interface that may be beyond our detection. It remains to be explored why only the very first layer is superconducting while the other layers above are not superconducting [1] . Clearly, the answer to these questions will provide crucial information on achieving even higher T c in searching for new high-temperature superconductors. Thin film preparation and post-annealing The single-layer FeSe thin films were grown on SrTiO 3 (001) substrate by the molecular beam epitaxy (MBE) method and were characterized by scanning tunnelling microscope. The details can be found in (ref. 1 ). To transfer the thin film sample from the MBE preparation chamber to a different ARPES measurement chamber, the prepared thin film is covered by an amorphous Se capping layer. The Se layer was desorbed by heating up the samples to 400 °C for 2 h before ARPES measurements. Sample temperature calibration Because the FeSe thin film on SrTiO 3 substrate is different from our usual cleaved sample, also owing to their different mounting methods on the cold finger of the cryostat, at the same temperature of the cold finger, the temperature on the FeSe thin film is higher than that for the usual cleaved sample. Therefore, the usual sample temperature sets a low limit to the temperature of the FeSe thin film. To measure the temperature of the FeSe thin film more accurately, we simulate the FeSe thin film by gluing a piece of polycrystalline gold foil on the similar SrTiO 3 substrate. By measuring the Fermi level of the gold from our high-resolution laser photoemission, we can measure the temperature of gold on SrTiO 3 from the gold Fermi level width fitted by the Fermi-distribution function. As the Fermi-level width contains a couple of contributions including the temperature broadening, instrumental resolution and cleanliness of gold, the estimated temperature sets an upper limit to the gold temperature that is close to the temperature of FeSe thin film on SrTiO 3 . We found the temperature measured from this gold reference is higher than the nominal usual sample temperature by ~10 K. The real temperature of the FeSe thin film then lies in between these two temperature limits, nominal sample temperature and gold temperature, with an error bar of ±5 K. High-resolution ARPES measurements High-resolution angle-resolved photoemission measurements were carried out on our lab system equipped with a Scienta R4000 electron energy analyzer [44] . We use helium discharge lamp as the light source that can provide photon energies of hυ= 21.218 eV (helium I). The energy resolution was set at 10 meV for the Fermi-surface mapping ( Fig. 1a ) and band-structure measurements ( Fig. 2 ) and at 4 meV for the superconducting gap measurements ( Figs 3 and 4 ). The angular resolution is ~0.3 degree. The Fermi level is referenced by measuring on a clean polycrystalline gold that is electrically connected to the sample. The sample was measured in vacuum with a base pressure better than 5×10 −11 Torr. How to cite this article: Liu, D. et al . Electronic origin of high-temperature superconductivity in single-layer FeSe superconductor. Nat. Commun. 3:931 doi: 10.1038/ncomms1946 (2012).